Electron–hole doping asymmetry of Fermi surface reconstructed in a simple Mott insulator It is widely recognized that the effect of doping into a Mott insulator is complicated and unpredictable, as can be seen by examining the Hall coefficient in high T c cuprates. The doping effect, including the electron–hole doping asymmetry, may be more straightforward in doped organic Mott insulators owing to their simple electronic structures. Here we investigate the doping asymmetry of an organic Mott insulator by carrying out electric-double-layer transistor measurements and using cluster perturbation theory. The calculations predict that strongly anisotropic suppression of the spectral weight results in the Fermi arc state under hole doping, while a relatively uniform spectral weight results in the emergence of a non-interacting-like Fermi surface (FS) in the electron-doped state. In accordance with the calculations, the experimentally observed Hall coefficients and resistivity anisotropy correspond to the pocket formed by the Fermi arcs under hole doping and to the non-interacting FS under electron doping. Electron–hole doping asymmetry in Mott insulators has been one of the key questions related to the origin of superconductivity in the proximity of the insulating state [1] , [2] , [3] . To investigate this, one should prepare an exactly half-filled (zero-doped) Mott insulator and then inject or extract electrons, preferably by an electrostatic method, in the same sample. However, it is difficult to perform such measurements on high- T c cuprates for the following three reasons. First, they are mostly either only hole-doped or electron-doped, and the crystallographic structures of the parent materials are often different. Second, they require a strong electric field to tune their band filling owing to their high half-filled carrier density (in the order of 10 15 cm −2 ). Third, since they are charge-transfer-type insulators, electrons and holes are doped into different electronic orbitals, which may obscure the pure doping asymmetry. In practice, the inverse of the Hall coefficient monotonically increases with increasing doping concentration with the sign changing across the zero-doping point [4] . This is a feature of band insulators rather than Mott insulators. In contrast to the high- T c cuprates, the organic Mott insulator κ -(BEDT-TTF) 2 Cu[N(CN) 2 ]Cl (ref. 5 ) (abbreviated to κ -Cl hereafter), where BEDT-TTF represents bis(ethylenedithio)tetrathiafulvalene, serves as an appropriate material for examining the electron–hole asymmetry of doped Mott insulators because of its relatively low carrier density ( ∼ 1.8 × 10 14 cm −2 ) and its single electronic orbital nature. Indeed, electrons and holes are doped into the same π electron band and thus κ -Cl can be modelled as a single-band Hubbard model on an anisotropic triangular lattice ( Fig. 1 ). Because of its high controllability of electronic states, κ -Cl has been studied intensively in terms of the bandwidth-controlled Mott transition between Mott insulating and superconducting states at half-filling [6] , [7] . The electrostatic method of carrier doping into organic Mott insulators with field-effect transistor (FET) structure has been implemented by the authors [8] , [9] . However, the limited doping concentration with the FET still forbids the observation of electron–hole asymmetry. 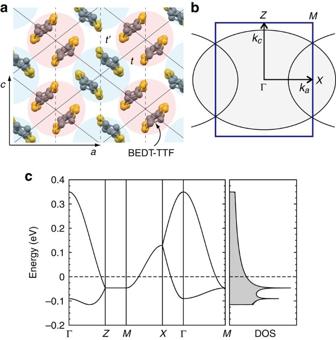Figure 1: Molecular arrangement and electronic structure ofκ-Cl without electron correlation. (a) Molecular arrangement of the BEDT-TTF layer and the effective anisotropic triangular lattice.tis the nearest-neighbour hopping (solid line) andt' is the next-nearest-neighbour hopping (dashed line) between the BEDT-TTF dimers. Two differently oriented dimers are indicated by red and blue shades. (b) Schematic representation of Fermi surface without electron interaction. The first BZ ofκ-Cl is indicated by a solid square. (c) Tight-binding band structure and DOS fort'/t=−0.8 witht=55 meV. Here, Γ=(0,0),Z=(0,π/c),M=(π/a,π/c) andX=(π/a,0). The Fermi energy is denoted by dashed lines. DOS, density of states. Figure 1: Molecular arrangement and electronic structure of κ -Cl without electron correlation. ( a ) Molecular arrangement of the BEDT-TTF layer and the effective anisotropic triangular lattice. t is the nearest-neighbour hopping (solid line) and t ' is the next-nearest-neighbour hopping (dashed line) between the BEDT-TTF dimers. Two differently oriented dimers are indicated by red and blue shades. ( b ) Schematic representation of Fermi surface without electron interaction. The first BZ of κ -Cl is indicated by a solid square. ( c ) Tight-binding band structure and DOS for t '/ t =−0.8 with t =55 meV. Here, Γ=(0,0), Z =(0, π / c ), M =( π / a , π / c ) and X =( π / a ,0). The Fermi energy is denoted by dashed lines. DOS, density of states. Full size image Here, by fabricating electric-double-layer transistors (EDLTs) based on thin single crystals of κ -Cl, we realized for the first time both electron and hole doping into the organic Mott insulator. We measured the field effect on transport properties including the sheet resistivity, Hall coefficient and resistivity anisotropy to elucidate the doping anisotropy of the electronic state in the doped organic Mott insulator. To provide further insights into the Fermi surface (FS), we calculated the single-particle spectral functions for an effective model of κ -Cl by using cluster perturbation theory (CPT) [10] , [11] . The calculations predict that strongly anisotropic suppression of the spectral weight results in the Fermi arc state under hole doping, while a relatively uniform spectral weight results in the emergence of a non-interacting-like FS in the electron-doped state. In accordance with the calculations, the experimentally observed Hall coefficients and resistivity anisotropy correspond to the pocket formed by the Fermi arcs under hole doping and to the non-interacting FS under electron doping. Resistivity We fabricated the EDLT devices by mounting an ion gel on a Hall-bar-shaped thin single crystal of κ -Cl and an Au-side gate electrode ( Fig. 2a,b ). First, we obtained the resistivity curve for the sheet resistivity ρ at the temperature T =220 K ( Fig. 2c ). As expected for a Mott insulator, a clear ambipolar field effect with a resistance peak at the gate voltage V g ≈−0.2 V was observed. The hysteresis and the leakage current remained small without any signature of a chemical reaction between the electrolyte and κ -Cl. Note that the field effect was ∼ 3% at 220 K, because thermally excited carriers in the bulk (about 100 molecular layers in a typical sample) dominated the electrical conduction owing to the low charge excitation gap ( ∼ 20 meV). We also confirmed that the carrier tunability of the κ -Cl EDLT greatly exceeded that of SiO 2 -based FETs by comparing these devices using the same κ -Cl crystal ( Supplementary Fig. 1 ). Provided that the mobilities of the FET and EDLT are equivalent, a gate voltage of +1 V in the EDLT corresponded to ∼ 20% electron doping (see Supplementary Note 1 ). The resistivity curves at 220 K and the temperature dependences of the resistivity were reproducible after multiple temperature cycles (see Supplementary Note 2 and Supplementary Fig. 2 ). 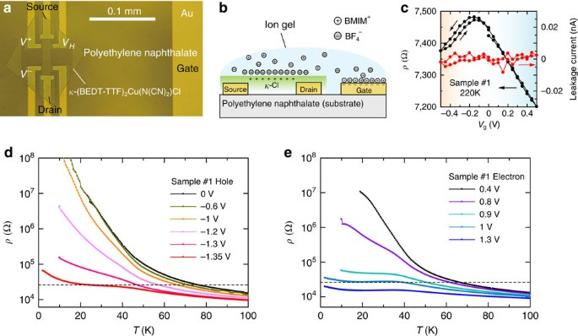Figure 2: EDLT device and field effect on sheet resistivity. (a,b) Optical top view (a) and schematic side view (b) of the EDLT device. Theκ-Cl crystal is shaped into a Hall-bar using a pulsed laser beam. (c) Gate voltage dependence of the sheet resistivity at 220 K. (d,e) Temperature dependence of the sheet resistivity under hole doping (d) and electron doping (e). The dashed lines denoteh/e2∼25.8 kΩ. The gate voltage was consecutively applied in the order of appearance, namely: 0, −0.6, −1, −1.2, −1.3 and −1.35 V for hole doping and 0.4, 0.8, 0.9, 1 and 1.3 V for electron doping. Figure 2: EDLT device and field effect on sheet resistivity. ( a,b ) Optical top view ( a ) and schematic side view ( b ) of the EDLT device. The κ -Cl crystal is shaped into a Hall-bar using a pulsed laser beam. ( c ) Gate voltage dependence of the sheet resistivity at 220 K. ( d,e ) Temperature dependence of the sheet resistivity under hole doping ( d ) and electron doping ( e ). The dashed lines denote h / e 2 ∼ 25.8 kΩ. The gate voltage was consecutively applied in the order of appearance, namely: 0, −0.6, −1, −1.2, −1.3 and −1.35 V for hole doping and 0.4, 0.8, 0.9, 1 and 1.3 V for electron doping. Full size image With decreasing temperature, the ambipolar field effect became more distinct. Figure 2d,e show the temperature dependence of the sheet resistivity under a negative gate voltage (hole doping) and positive gate voltage (electron doping), respectively. Under hole doping, the activation energy significantly decreased to <1 meV at V g =−1.35 V. On the other hand, the doping of electrons tended to reduce the resistivity more effectively and metallic conductivity was observed at V g >1 V. In a high-conductivity sample, we observed negative magnetoresistance accompanied with the upturn of resistivity at low temperature, which suggested a weak localization effect (see Supplementary Note 3 and Supplementary Fig. 3 ). Analysis of the weak localization indicated that the mean free path and dephasing length considerably exceeded the distance between BEDT-TTF dimers indicating coherent transport. Hall effect To observe a more significant difference between the electron- and hole-doped states, we measured the Hall coefficient R H , which indicates the FS topology. The magnetic field B dependence of the Hall resistance R xy at 30 K is shown in Fig. 3a ( R H is given by the slope). Despite electron doping, the Hall coefficients were clearly positive and a simple estimation of the carrier density, 1/ eR H , gave ∼ 0.8 holes per BEDT-TTF dimer. Since the injected carriers were electrons ( ∼ 0.2 electrons/dimer), the concentration of which was much lower than that of the observed holes, it suggests that dense hole carriers are delocalized by electron doping. This is considered to be the doping-induced Mott transition previously observed in FET devices [12] . 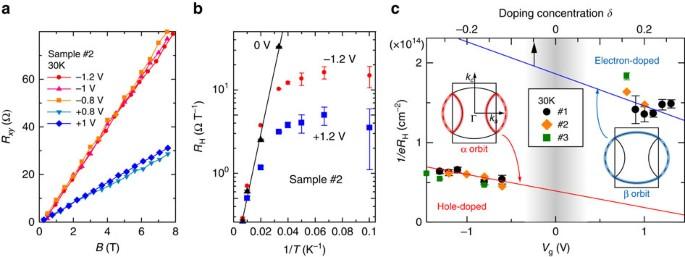Figure 3: Hall effect. (a) Hall resistance versus magnetic field at 30 K. (b) Temperature dependence ofRHatVg=−1.2, 0 and +1.2 V. The solid line represents the fit 8.78 × 10−2× exp (Ea/kBT) ΩT−1with an activation energyEa/kB=176 K to the data of the undoped bulk crystal. The error bars were calculated from the s.d. of the Hall resistance versus magnetic field plots. Note that the data below 25 K contain further errors owing to the non-ohmic behaviour (Supplementary Note 6). (c) Gate voltage dependence of 1/eRHat 30 K. Data from three different samples are shown. The solid lines denote the 1/eRHestimated from the volume bounded by the non-interacting FS (blue) and by the lens-like closed portion of the FS (red). Namely, the blue and red solid lines represent densities of the total carriers and the partial carriers enclosed by the lens-like closed portion, respectively. Here, the electron doping concentrationδis related to the non-interacting hole densityn(=1−δ) which is evaluated for the anisotropic Hubbard model withU=0. On the basis of the FET and EDLT measurements, the top horizontal axis is set in thatδ=0.2 corresponds toVg=1 V (seeSupplementary Note 1). Figure 3: Hall effect. ( a ) Hall resistance versus magnetic field at 30 K. ( b ) Temperature dependence of R H at V g =−1.2, 0 and +1.2 V. The solid line represents the fit 8.78 × 10 −2 × exp ( E a / k B T ) ΩT −1 with an activation energy E a / k B =176 K to the data of the undoped bulk crystal. The error bars were calculated from the s.d. of the Hall resistance versus magnetic field plots. Note that the data below 25 K contain further errors owing to the non-ohmic behaviour ( Supplementary Note 6 ). ( c ) Gate voltage dependence of 1/ eR H at 30 K. Data from three different samples are shown. The solid lines denote the 1/ eR H estimated from the volume bounded by the non-interacting FS (blue) and by the lens-like closed portion of the FS (red). Namely, the blue and red solid lines represent densities of the total carriers and the partial carriers enclosed by the lens-like closed portion, respectively. Here, the electron doping concentration δ is related to the non-interacting hole density n (=1− δ ) which is evaluated for the anisotropic Hubbard model with U =0. On the basis of the FET and EDLT measurements, the top horizontal axis is set in that δ =0.2 corresponds to V g =1 V (see Supplementary Note 1 ). Full size image If we assume doping symmetry, a similar Hall effect is expected for the hole-doped side. Namely, hole doping immediately collapses the Mott–Hubbard gap and 1/ eR H corresponding to 1− δ ( δ : electron doping concentration, which is negative for hole doping) holes per BEDT-TTF dimer should be observed. However, as shown in Fig. 3a , the Hall coefficient on the hole-doped side was about three times larger than that on the other side, and 1/ eR H gave ∼ 0.3 holes per BEDT-TTF dimer. Although 1/ eR H increased with increasing absolute value of the gate voltage, the rate of increase was low (only 7% difference between V g =−0.8 V and −1.2 V). Surprisingly, under hole doping, 1/ eR H per dimer appears to be neither 1− δ (delocalized hole carriers+injected hole carriers) nor− δ (only injected hole carriers), indicating that the localized carriers were partially delocalized by excess hole doping as shown in Fig. 3c . These results indicate that the FS topology is significantly different between the electron- and hole-doped states. For the gate voltage dependence of the Hall mobility, see Supplementary Note 4 and Supplementary Fig. 4 . The temperature dependence of R H ( Fig. 3b ) shows that the R H asymmetry was maintained up to ∼ 50 K, above which the Hall effect at the doped surface was obscured by the thermally excited carriers in the bulk. Note that increase in R H at 30 K upon cooling is due to the decrease of the thermally excited carriers in the bulk (see Supplementary Note 5 and Supplementary Fig. 5 ). The data below 25 K contain ambiguity owing to the non-ohmic behaviour (see Supplementary Note 6 and Supplementary Fig. 6 ). What is the origin of R H under hole doping? As shown in Fig. 1 , κ -Cl forms essentially an anisotropic triangular lattice resulting in an ellipsoidal non-interacting FS which is folded by the zone boundary. In a Fermi liquid with a single type of carrier, 1/ eR H denotes the carrier density corresponding to the volume enclosed by the FS (Luttinger’s theorem [13] ). Under electron doping, 1/ eR H is close to the carrier density corresponding to the non-interacting ellipsoidal FS (known as the β -orbit in the study of Shubnikov-de Haas oscillation [14] ). By contrast, 1/ eR H under hole doping somehow appears to correspond to the volume bounded by the lens-like closed portion of the FS (known as the α -orbit). The doping dependences of the carrier density enclosed by the α - and β -orbits assigned for a κ -BEDT-TTF salt [15] are plotted as reference in Fig. 3c . Single-particle spectral functions To verify this R H asymmetry, we calculated the single-particle spectral functions of the Hubbard model on an anisotropic triangular lattice ( t ′/ t =−0.8, U / t =7) at 30 K using CPT and the results are shown in Fig. 4 . First, the Mott insulating state was reproduced at half-filling, where the energy gap opened at all the k-points ( Fig. 4b,e ). When electrons were doped ( δ =+0.17), the FS appeared as shown in Fig. 4c,f . The FS topology was the same as that of the non-interacting case, although the shape and the spectral weight were not exactly the same. In this state, the value of R H should be close to that of the Fermi liquid state, as suggested by the experiments. On the other hand, the FS under hole doping ( δ =−0.17) was very different from the non-interacting FS ( Fig. 4a,d ). The spectral weight near the Z point was strongly suppressed. Namely, arcs around the X point and pseudogaps near the Z point appeared. The partial disappearance of FS by the pseudogap is similar to the Fermi arc state observed in lightly hole-doped cuprates [16] , [17] , [18] . In this state, Luttinger’s theorem is seemingly violated and the value of R H is no longer simply estimated. However, considering the first Brillouin zone (BZ) of κ -Cl, one can see that the Fermi arcs are folded and form closed lens-like orbits. These orbits originate from the α -orbit mentioned above and correspond to the observed R H in the hole-doped states. These results imply that R H is predominantly governed by quasi-particles with relatively long lifetime (bright points of the spectral function in the reciprocal space in Fig. 4 ). Therefore, the asymmetry of the FS topology was clearly observed via R H . 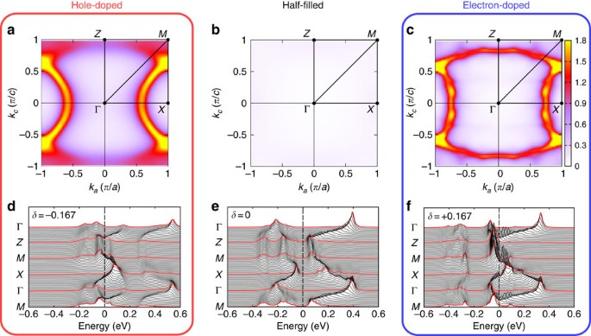Figure 4: Fermi surfaces and the single-particle spectral functions of the Hubbard model on an anisotropic triangular lattice at 30 K. (a–c) Fermi surfaces in the first BZ ofκ-Cl for 17% hole doping (a), half-filling (b) and 17% electron doping (c), determined by the largest spectral intensity at the Fermi energy. (d–f) Single-particle spectral functions for 17% hole doping (d), half-filling (e) and 17% electron doping (f). The Fermi energy is located atω=0 and the parameter set of this model ist'/t=−0.8,U/t=7 andt=55 meV. Figure 4: Fermi surfaces and the single-particle spectral functions of the Hubbard model on an anisotropic triangular lattice at 30 K. ( a – c ) Fermi surfaces in the first BZ of κ -Cl for 17% hole doping ( a ), half-filling ( b ) and 17% electron doping ( c ), determined by the largest spectral intensity at the Fermi energy. ( d – f ) Single-particle spectral functions for 17% hole doping ( d ), half-filling ( e ) and 17% electron doping ( f ). The Fermi energy is located at ω =0 and the parameter set of this model is t '/ t =−0.8, U / t =7 and t =55 meV. Full size image Anisotropy of the resistivity The partial disappearance of the FS can also be confirmed by the anisotropy in the carrier conduction. The strongly suppressed parts of the FS under hole doping should affect strongly the carrier conduction along the c axis. Indeed, our CPT calculations predict that the resistivity is more anisotropic in the hole-doped state than in the electron-doped state (see Supplementary Note 7 and Supplementary Fig. 7 ). We measured the resistivity anisotropy as shown in Fig. 5 . The crystallographic axes were determined by the crystal shape and the sign of the Seebeck coefficient at room temperature. At 220 K, where the thermally excited carriers in the non-doped bulk dominate the conductivity, the c axis resistivity ρ c was slightly higher than the a axis resistivity ρ a in both electron and hole doping. With decreasing temperature ρ c / ρ a increased under hole doping, while it decreased and remained near 1 in the non-doped and electron-doped states as shown in Fig. 5b . The contour plot of ρ c / ρ a under various gate voltage and temperature ( Fig. 5c ) clearly exhibited that the resistivity in the hole-doped state was particularly anisotropic, in good qualitative agreement with our CPT calculations. 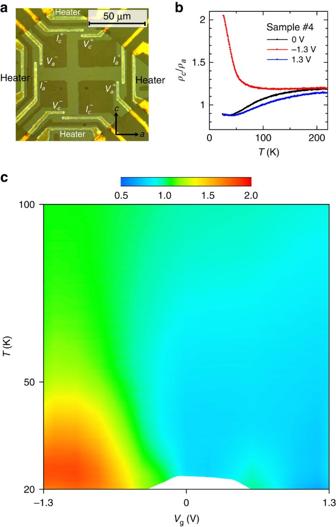Figure 5: Anisotropy of the resistivity. (a) Optical image of the sample. The crystallographic axes were assigned by the heat measurement because theaaxis (caxis) shows positive (negative) Seebeck coefficient at room temperature. (b) Temperature dependence ofρc/ρaatVg=−1.3, 0 and +1.3 V. Here,ρc(ρa) is the resistivity along thecaxis (aaxis). (c) Contour plot ofρc/ρaas a function ofTandVg. The applied gate voltages were −1.3, −1.2, −1, −0.8, −0.6, −0.4, −0.2, 0, 0.2, 0.4, 0.6, 0.8, 1, 1.2 and 1.3 V. Data are missing at low temperature and low doping (white region) due to the high resistance. Figure 5: Anisotropy of the resistivity. ( a ) Optical image of the sample. The crystallographic axes were assigned by the heat measurement because the a axis ( c axis) shows positive (negative) Seebeck coefficient at room temperature. ( b ) Temperature dependence of ρ c / ρ a at V g =−1.3, 0 and +1.3 V. Here, ρ c ( ρ a ) is the resistivity along the c axis ( a axis). ( c ) Contour plot of ρ c / ρ a as a function of T and V g . The applied gate voltages were −1.3, −1.2, −1, −0.8, −0.6, −0.4, −0.2, 0, 0.2, 0.4, 0.6, 0.8, 1, 1.2 and 1.3 V. Data are missing at low temperature and low doping (white region) due to the high resistance. Full size image The doping asymmetry is expected from the particle–hole asymmetric non-interacting band structure, as shown in Fig. 1c . The energy bands along the Z–M axis are very flat and the van Hove singularity (vHs) lies below the FS at half-filling. With the doping of holes, the FS approaches the vHs and the effect of the interaction is expected to be enhanced. Indeed, substantial suppression of the spectral weight of the FS along the Z–M axis, on which the van Hove critical points lie, is observed ( Fig. 4a ). By contrast, the FS departs from the vHs with the doping of electrons, resulting in a weaker interaction effect and a more non-interacting-like FS. It is also indicated that the spin fluctuation is stronger in the hole-doped state because of the vHs. If a superconducting state could be induced by further hole doping, the transition temperature and pairing symmetry are of great interest since the hole-doped state is substantially different from the metallic state created by controlling the bandwidth at half-filling. To summarize, without gate voltage, κ -Cl is a Mott insulator due to electron interaction and high commensurability between the hole density and periodic potential (one hole/one site). When holes or electrons are doped, the commensurability is reduced and the effect of electron interaction is weakened, resulting in carrier delocalization. However, the effect of interaction remains strong at specific k-points where the energy dispersion is relatively flat. Owing to the particle–hole asymmetric band structure, the pseudogaps appeared only near the van Hove critical points under hole doping. In contrast to the calculations, our measurements did not observe the true metallic state (d ρ /d T >0) at low temperature. This is probably due to the effect of localization caused by finite random potential at the surface [19] , [20] , as the negative magnetoresistance indicated. Improvement of the surface roughness and cleanness may realize metallic phases under both dopings. Thus, the doping asymmetry in a Mott insulator was demonstrated by a simple process in an organic Mott EDLT. The above results show that organic Mott insulators are good model materials for Mott physics even in the case of band-filling control, and the electronic state in a simple Mott insulator may be predictable in the framework of CPT. Since molecular conductors consist of various molecules with different arrangements, the effect of doping into materials with different FS topologies is of interest in future experiments. Furthermore, the presence/absence of the superconducting phase under doping and its doping asymmetry are also intriguing. Sample preparation The source, drain and gate electrodes (18 nm thick Au) were patterned on a polyethylene naphthalate substrate (Teonex Q65FA, Teijin DuPont Films Japan Limited) using photolithography. A thin ( ∼ 100 nm) single crystal of κ -(BEDT-TTF) 2 Cu[N(CN) 2 ]Cl (abbreviated to κ -Cl hereafter) was electrochemically synthesized by oxidizing BEDT-TTF (20 mg) dissolved in 50 ml of 1,1,2-trichloroethane (10% v/v ethanol) in the presence of TPP[N(CN) 2 ] (TPP, tetraphenylphosphonium; 190 mg), CuCl (60 mg) and TPP-Cl (100 mg). After applying current of 8 μA for 20 h, a thin crystal was transferred into 2-propanol with a pipette and was guided on top of the PEN substrate. After the substrate was removed from the 2-propanol and dried, the κ -Cl crystal was shaped into a Hall-bar using a pulsed laser beam with a wavelength of 532 nm. Typical dimensions of the Hall bar sample were approximately 15 μm (width) × 40 μm (length) × 100 nm (thickness). The EDLT devices were completed by mounting an ion gel (or ionic liquid) on the Hall-bar-shaped thin single crystal of κ -Cl and an Au-side gate electrode. The basic techniques, such as the electrochemical synthesis of thin single crystals and the laser shaping, are common to our previous FET devices [12] . As gate electrolytes, we employed poly(vinylidene fluoride-co-hexafluoropropylene) (PVDF-HFP) with 58% w/w 1-butyl-3-methylimidazolium tetrafluoroborate (BMIM-BF 4 ) (samples #1 ∼ 4), N,N-diethyl-N-methyl-N-(2-methoxyethyl) ammonium bis(trifluoromethanesulfonyl)imide (DEME-TFSI) (sample #5 in Supplementary Fig. 1 ), polymethyl methacrylate (PMMA) with 57% w/w DEME-TFSI (sample #6 in Supplementary Fig. 3 ). The PVDF-HFP ion gel [21] was spin-coated from an acetone solution in which the weight ratio between the polymer, ionic liquid and solvent was 1:1.3:7.7. Although the ionic conductivity was the greatest in the liquid state, the large thermal stress usually broke the κ -Cl crystal at a low temperature ( T <150 K). Thinning of the gate electrolytes by gelation reduced the thermal stress at low temperatures, allowing the successful cooling of the samples down to 2 K. The area of the gate electrode was more than 100 times larger than that of the κ -Cl channel in order to apply the gate voltage effectively. Transport measurements The transport measurements were performed using a Physical Property Measurement System (Quantum Design). The temperature and magnetic field normal to the substrate were controlled in the range of 2–300 K (cooling rate: 2 K min −1 ) and ±8 T, respectively. When the gate voltage was varied, the samples were warmed to 220 K. In the Hall measurements, the magnetic field was swept in the range of ±8 T at a constant temperature and the forward and backward data were averaged to eliminate the small linear voltage drift. Although it is difficult to experimentally determine the distribution of field-induced charge along the out-of-plane direction, we consider that the field-induced carriers predominantly exist in a single conducting molecular sheet [12] . Recently, the quantum oscillations in the doped surface of the Dirac fermion system α -(BEDT-TTF) 2 I 3 (ref. 22 ) indicated that only two conducting layers from the surface were doped, in which the carrier density in the second layer was only 1/7 of that in the first layer. The above assumption is also likely to apply to κ -type BEDT-TTF salts, where a shorter screening length is expected. Hubbard model on an anisotropic triangular lattice To examine the electron correlation effects in the organic doped Mott insulator, we study the single-band Hubbard model defined on an anisotropic triangular lattice, which is known as the simplest model for κ -type BEDT-TTF salts [23] , [24] , [25] , [26] . The model is defined by the Hamiltonian where creates an electron on site i with spin σ (=, ) and . t ij is the transfer integral between the neighbouring sites i and j , U is the on-site Coulomb repulsion and μ is the chemical potential. Here, a single site consists of a single dimer and a unit cell contains two dimers with different orientation ( Supplementary Fig. 8a ). The transfer integral between the different (same) dimers is given as t ij = t ( t ′). The series of κ -type BEDT-TTF salts serves as an ideal realization of the Hubbard model of equation (1). The anisotropy | t ′/ t | can be changed depending on substituted anions [26] , [27] , [28] , [29] . The Coulomb repulsion U is estimated to be comparable to [29] , [30] or larger than [26] the band width, implying that the strongly correlated electronic state is realized at ambient pressure. Applied pressure [28] , [31] , [32] or bending strain on thin films [33] can control the electron correlation parameter t / U . Moreover, the chemical potential μ can be tuned efficiently by applied gate voltage in the EDLT, allowing for investigation of the electronic structure of electron- and hole-doped Mott insulators on equal footing. The series of organic charge transfer salts is indeed the highly controllable counterpart of strongly correlated transition-metal compounds [34] . In the main text, we have focused on a typical parameter set for κ -type BEDT-TTF salts of t ′/ t =−0.8, U / t =7 and t =55 meV. We have also considered the parameter set relevant for κ -Cl of t ′/ t =−0.44, U / t =5.5 and t =65 meV (ref. 29 ), and found that the Fermi arc appears for hole-doped case also in this parameter set ( Supplementary Fig. 9 ). The non-interacting tight-binding band structure, the density of states, and the FS at half-filling for this parameter set are shown in Supplementary Fig. 8c,d . The strongly correlated Hubbard model at half-filling or the Heisenberg model on the anisotropic triangular lattice have been investigated theoretically and the ground-state phase diagrams with various phases including metal, anti-ferromagnetic insulator, spiral, and spin liquid ground states have been obtained [35] , [36] , [37] , [38] , [39] , [40] , [41] , [42] . Most of these previous calculations on the Hubbard model at half-filling have been carried out with t ′/ t >0. However, the sign of t ′ is crucial when it comes to the electron–hole asymmetry of carrier doping because the sign determines whether the vHs appears in hole-doped side or electron-doped side. The correct sign is t ′/ t <0 (ref. 26 ) and the vHs appears in the hole-doped side (see Fig. 1c and Supplementary Fig. 8c ). Unit cell and Brillouin zone In Fig. 4 and Supplementary Fig. 9 , we show the single-particle spectral functions and the FSs in the BZ of the unit cell consisting of two sites in the real space (see blue shaded region in Supplementary Fig. 10a ). The BZ is relevant for the realistic structure of the κ -type BEDT-TTF salts and therefore the results are directly compared with those obtained by first-principles band-structure calculations [26] , [29] . However, the primitive unit cell of the single-band Hubbard model in equation (1) on the anisotropic triangular lattice consists of one site (see red shaded region in Supplementary Fig. 10a ), unless a spontaneous symmetry breaking such as the Néel order occurs. Therefore the theoretical calculations for the Hubbard model on the anisotropic triangular lattice are usually performed with this primitive unit cell [36] , [37] , [38] , [39] , [40] , [41] , [42] , [43] . In order to avoid possible confusions caused by the different choice of the unit cell, we describe the relation between the two BZs of the one-site unit cell and the two-site unit cell. Supplementary Figure 10a shows the anisotropic triangular lattice with regular-triangular plaquettes. The primitive translational vectors for the one (two)-site unit cell are given by { e 1 , e 2 } ({ a , c }), and the corresponding BZ is diamond (rectangular) shaped, as shown in Supplementary Fig. 10c . We also show in Supplementary Fig. 10b the lattice which is topologically equivalent to the triangular lattice in Supplementary Fig. 10a but forms the square plaquettes with diagonal lines. Notice that this square topology of the lattice is very often used for study of the Hubbard model on the anisotropic triangular lattice [36] , [37] , [38] , [39] , [40] , [43] . The primitive translational vectors for the one (two)-site unit cell are again given by { e 1 , e 2 } ({ a , c }). The BZ of the one (two)-site unit cell is now square (diamond) shaped, as shown in Supplementary Fig. 10d . Let us now consider the basis-transformation formula between the bases { a , c } and { e 1 , e 2 }, where the former is a set of the primitive translational vectors of the realistic structure of the κ -type BEDT-TTF salts, while the latter is that of the single-band Hubbard model. It is easily found from Supplementary Fig. 10b that they are related by the ± π /4 rotation and the scale transformation. To be concrete, we consider a vector r = r a a + r c c = r 1 e 1 + r 2 e 2 in the real space. It is easily shown that the coordinate ( r a , r c ) is related to the coordinate ( r 1 , r 2 ) as Similarly, for a wave vector k = k a g a + k c g c = k 1 g 1 + k 2 g 2 , where {2 π g a , 2 π g c } ({2 π g 1 , 2 π g 2 }) is the set of the reciprocal vectors of { a , c } ({ e 1 , e 2 }), ( k a , k c ) is related to ( k 1 , k 2 ) as For example, ( k a , k c )=(0, 0),(0, π ),( π , π ) and ( π , 0) in the { g a , g c } basis (that is, Γ, Z , M and X points in Supplementary Fig. 10c ) correspond to ( k 1 , k 2 )=(0, 0),( π /2, π /2), ( π , 0) and ( π /2, − π /2) in the { g 1 , g 2 } basis ( Supplementary Fig. 10d ), respectively. Finally, we note that the rectangular BZ in Supplementary Fig. 10c corresponds to the anti-ferromagnetic BZ of the square lattice in Supplementary Fig. 10d (blue shaded regions). Cluster perturbation theory To examine the electron–hole asymmetry of the FS, the calculation of single-particle Green’s functions is required. For this purpose, we employ the CPT [11] . The CPT is a theory of strong coupling expansion for the single-particle Green’s function and allows us to examine the single-particle excitations including quasi-particle excitations, Mott gap, and even pseudogap phenomena in strongly correlated electron systems [43] , [44] , [45] . As shown in the following, the CPT requires the fully interacting single-particle Green’s function (or the self-energy [46] , [47] ) of open-boundary clusters to obtain the single-particle Green’s function of the lattice. The basic notion of the scheme was introduced in the earlier work by Gros and Valentí [10] . Let us outline the method of CPT. First, we divide the whole lattice on which the model Hamiltonian H is defined into identical finite-size clusters, each of which consists of L c sites. We shall denote the Hamiltonian of a cluster as and the inter-cluster hopping as . Here, is given in the right-hand side of equation (1) but it is defined on a L c -site cluster with open-boundary conditions. Next, the single-particle Green’s function G c of the cluster Hamiltonian is calculated by the exact diagonalization method. Applying the strong coupling expansion with respect to the inter-cluster hopping , the single-particle Green’s function is given as , where is the matrix representation of (ref. 48 ). By restoring the translational invariance, which is broken in due to the partitioning of the lattice, we obtain the single-particle Green’s function G of the whole lattice for momentum k and complex frequency z as where r i is the position of the i -th site within the cluster [48] . The cluster Green’s function matrix G c is given as with and where β =1/ k B T with T being the temperature, |Ψ s 〉 is the s -th eigenstate of with its eigenvalue E s in ascending order, and is the partition function of the cluster. The sum over eigenstates is truncated by summing up to the s max -th eigenstate. The upper bound s max of the sum is determined so as to satisfy that , where E 0 is the ground-state energy and is a small real number. For the finite temperature calculations at T =100 K, we set , in which for example the lowest s max ∼ 1,400 eigenstates among 4 12 eigenstates in total are included for the hole-doped case with L c =12. The inter-cluster hopping between different clusters in equation (4) is represented as where t ij is given in equation (1), X 1 and X 2 are the translational vectors of the clusters, and m 1 X 1 + m 2 X 2 ( m 1 and m 2 : integer) indicates a relative position of two different clusters, site i being located in one cluster and site j in the other cluster. For the 12-site cluster, the translational vectors are X 1 =2.5 a +0.5 c and X 2 =0.5 a +2.5 c , and t ij in equation (8) is finite only when ( m 1 , m 2 )=(±1, 0), (0, ±1) and (±1, ±1), indicating the inter-cluster hopping between a cluster and its neighbouring six clusters (see Supplementary Fig. 8a ). For the 16-site cluster, the translational vectors are X 1 =2 a +2 c and X 2 =−2 a +2 c , and t ij in equation (8) is finite only when ( m 1 , m 2 )=(±1, 0), (0, ±1), and (±1, ±1) (see Supplementary Fig. 8b ). Note that in principle a cluster with a larger size gives better results in the CPT because the electron correlation effects including spatial fluctuations within a cluster are fully taken into account. We have shown in the main text and Supplementary Fig. 9 the single-particle spectral functions using the 12-site cluster at finite temperatures. We also show in Supplementary Figs 11 and 12 the single-particle spectral functions for the 16-site cluster at zero temperature (see also Supplementary Note 8 ), where s max =0 in equations (6) and (7). The results clearly demonstrate that the electron–hole asymmetric reconstruction of the FS is observed irrespectively of the cluster sizes used. As a technical point, we have made use of the C 2 v symmetry of the 12- and 16-site clusters to reduce computational costs for solving the eigenvalue problem of and for calculating the cluster single-particle Green’s functions. Single-particle spectral function As shown in Supplementary Fig. 8a , the partitioning of the triangular lattice into the 12-site clusters does not respect the C 2 v symmetry (for lack of the σ v reflection symmetry) and the two-site unit cell structure (as X 1 and X 2 connect differently oriented dimers) of the dimer model on the anisotropic triangular lattice. However, these can be restored by averaging the single-particle Green’s functions over four different momenta, that is, This is because the average of the Green’s functions between k =( k a , k c ) and (− k a , k c ) restores the σ v reflection symmetry and the addition of the Green’s functions with wave vectors shifted by a primitive reciprocal vector, that is, k =(± k a , k c +2 π / c ), recovers the two-site unit cell structure in the BZ. Therefore, given in equation (9) provides the single-particle Green’s function relevant for the Hubbard model defined on the anisotropic triangular lattice even with the 12-site cluster. On the other hand, partitioning of the lattice into the 16-site clusters respects both the C 2 v symmetry and the two-site unit cell structure (see Supplementary Fig. 8b ). Therefore, the single-particle Green’s function with 16-site cluster is calculated in a standard way of the CPT for multi-band models described in ref. 48 . Using , the single-particle spectral function is calculated as where a small imaginary part i η of the complex frequency gives the Lorentzian broadening of the spectra. The FS is determined with the single-particle spectral function at zero energy, A ( k ,0). We set the Lorentzian broadening factor η / t =0.2 for the single-particle spectral functions and η / t =0.15 for the FS calculation. The single-particle spectral functions and FS are shown in Fig. 4 and Supplementary Figs 11 and 12 ( t ′/ t =−0.8, U / t =7 and t =55 meV), and in Supplementary Fig. 9 ( t ′/ t =−0.44, U / t =5.5 and t =65 meV). Data Availability The data that support the findings of this study are available from the corresponding authors upon request. How to cite this article: Kawasugi, Y. et al . Electron–hole doping asymmetry of Fermi surface reconstructed in a simple Mott insulator. Nat. Commun. 7:12356 doi: 10.1038/ncomms12356 (2016).